Engineering human tumour-associated chromosomal translocations with the RNA-guided CRISPR–Cas9 system Cancer-related human chromosomal translocations are generated through the illegitimate joining of two non-homologous chromosomes affected by double-strand breaks (DSB). Effective methodologies to reproduce precise reciprocal tumour-associated chromosomal translocations are required to gain insight into the initiation of leukaemia and sarcomas. Here we present a strategy for generating cancer-related human chromosomal translocations in vitro based on the ability of the RNA-guided CRISPR–Cas9 system to induce DSBs at defined positions. Using this approach we generate human cell lines and primary cells bearing chromosomal translocations resembling those described in acute myeloid leukaemia and Ewing’s sarcoma at high frequencies. FISH and molecular analysis at the mRNA and protein levels of the fusion genes involved in these engineered cells reveal the reliability and accuracy of the CRISPR–Cas9 approach, providing a powerful tool for cancer studies. Recurrent reciprocal chromosomal translocations are one of the most common types of genetic rearrangements and are considered primary causes of many cancers. They are present in more than 50% of all haematological malignancies and many have also been identified in sarcomas and in some epithelial tumours [1] . Chromosomal translocation in vivo is a complex biological process triggered by the simultaneous occurrence of DNA double-strand breaks (DSBs) at two loci of non-homologous chromosomes, followed by their illegitimate joining [2] , [3] . One consequence of this is the generation of oncogenic fusion genes. The genetic and molecular effects of these fusion genes have been extensively investigated in patient-derived cell lines. However, these cell lines do not recapitulate the initial steps of cancer development in vivo because they accumulate secondary mutations already present in the primary tumour cells and alterations in their gene expression profiles derived from extended periods in culture. There is therefore a need for more accurate models. Several strategies have been used to mimic the effects of the fusion protein, the most accurate approach being to experimentally generate a chromosomal translocation. Mouse chromosomal translocations with predetermined breakpoints were first created using Cre/loxP recombination [4] , [5] . More recently, with new engineering tools, zinc finger (ZFN) and transcription activator-like effector (TALEN) nucleases have been used to engineer de novo translocation in human cells [1] , [6] . The repertoire of genome engineering tools has recently expanded with the inclusion of the clustered regularly interspaced short palindromic repeats (CRISPR) and the associated Cas9 nucleases. These programmable RNA-guided endonucleases (RGEN) are composed of two RNA elements, the CRISPR RNA (cRNA) and its transactivating RNA (tracRNA), which can be fused together through a linker sequence to provide greater flexibility both in the design and applicability of this technology [7] . The CRISPR–Cas9 system has been applied into a variety of gene modification processes in human cells, including targeted genome engineering [8] , [9] , transactivation and silencing module factors [10] , and genetic correction [11] , and has even been used as a platform to induce large chromosomal deletions or inversions [9] , [12] . However, to our knowledge CRISPR–Cas9 technology has not yet been adapted to generate human chromosomal translocations. As indicated above, the generation of chromosomal translocations is assumed to be triggered by the formation of DSBs [13] , and we therefore reasoned that the introduction of concurrent DSBs at defined loci using the CRISPR/Cas9 system might induce reciprocal translocation between non-homologous chromosomes. As test models we chose two cancers of different origin that are defined by the occurrence of chromosomal translocations: Ewing’s sarcoma (ES) and acute myeloid leukaemia (AML). ES is a rare aggressive tumour that occurs primarily in children, adolescents and young adults and that typically arises in tissues of mesenchymal origin. Its chromosomal hallmark is the t(11;22)(q24;q12) chromosomal translocation, which leads to the generation of the EWSR1–FLI1 fusion gene [14] . The other cancer we selected is AML, a heterogeneous group of haematopoietic disorders characterized by the abnormal proliferation of immature myeloid progenitor cells with incapacity to differentiate [15] . AML patients with the cytogenetic t(8;21)(q22;q22) abnormality represent a subset with specific clinical and biological characteristics [16] . The translocation fuses the RUNX1 gene on chromosome 21 with the ETO gene on chromosome 8. Full elucidation of the pathogenesis of these cancers requires understanding of the tumour-initiating programme induced by the fusion proteins. We report a new approach to trigger defined chromosomal translocations using the CRISPR–Cas9 system. The establishment of cellular models of human chromosomal translocation will allow not only identification of the causative mutations required for malignant transformation but also screening of candidate drugs for patient treatment. For our models, we used two chromosomal translocations characteristic of malignancies of mesenchymal and haematopoietic origin. The translocations were induced in the human embryonic kidney (HEK) 293A cell line and in human mesenchymal and haematopoietic stem cells. The frequencies obtained indicate that this is a robust and efficient strategy for modelling the effects of rearrangements produced by chance in cancer cells. Induction of ES t(11;22) chromosomal translocation For our first test model of the induction of chromosomal translocation we chose ES. ES is characterized by the t(11;22)(q24;q12) chromosomal translocation, which leads to the generation of the EWSR1–FLI1 fusion gene [14] . Many alternative forms of EWS-FLI1 exist because of variations in the locations of the EWS and FLI1 genomic breakpoints. The most common form, designated ‘type 1’, consists of the first seven exons of EWS joined to exons 6–9 of FLI1 and accounts for ~60% of cases. The ‘type 2’ EWS–FLI1 fusion also includes FLI1 exon 5, and is present in 25% of cases. These forms are associated with different clinical features and prognoses [17] . 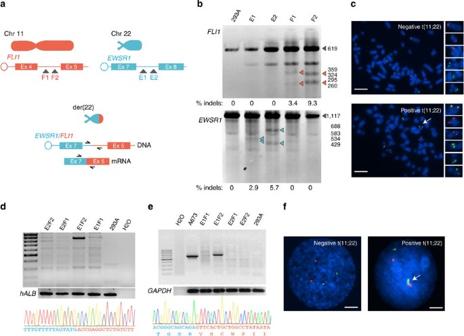Figure 1: Chromosomal translocation between theEWSR1andFLI1loci, mediated by CRISPR/Cas9 and sgRNA. (a) The translocation strategy. DSBs are introduced by the sgRNAs (arrowheads) mapping to introns inFLI1(orange) andEWSR1(turquoise). (b) Double-strand breaks in the targeted loci were generated by transfection of HEK293A cells with a plasmid expressing the Cas9 gene and sgRNAs E1, E2, F1 or F2. Grey arrowhead marks undigested PCR product; orange (FLI1) or turquoise (EWSR1) arrowheads mark digested products. Numbers on the right indicate the band sizes. The percentage of DSB is shown for each sgRNA (% indels), calculated as described in the Methods section. 293A, control non-transfected HEK293 cells. (c) Recovery of t(11:22) translocation after transfection with E1F2 sgRNAs. FISH analysis with theEWSR1single-fusion probe (green, chr22; red chr11) verified reciprocal translocation (yellow signals, arrow) on representative metaphase spreads of transfected HEK293 cultures with sgRNA E1F2 and CRSIPR/Cas9. For a detailed data set seeSupplementary Table 2. Scale bars represent 10 μm (d) Genomic PCR analysis to identify translocation breakpoint junctions. The positions of the primers used for PCR are indicated by angle symbols in the scheme in (a). The sequence of the amplified band is presented in the retrieved chromatogram at the bottom. 293A, non-transfected HEK293 cells. PCR control (bottom lane); detection of single copy albumin gene. (e) RT–PCR analysis ofEWSR1–FLI1fusion transcript expression in hygromycin-selected HEK293 cells. The positions of the primers used for PCR are indicated by angle symbols in the scheme in (a). The sequence of one representative clone is shown at the bottom. PCR control (bottom lane); detection of GAPDH. A673, ES cell line. (f) FISH analysis showingEWSR1translocation in human MSCs. Interphase nuclei are depicted with colour probes as in (c). Scale bars represent 5 μm. To target the more aggressive ‘type 2’ subtype [18] , we selected four small guide (sg) RNAs ( Supplementary Table 1 ) according to published criteria [19] that map to intron 4 (F1 and F2) in FLI1 and intron 7 (E1 and E2) in EWSR1 ( Fig. 1a ). To test the efficiency of each sgRNA in inducing specific DSBs at its defined location, we co-transfected HEK293A cells with the sgRNA-expressing plasmid and a plasmid expressing the optimized codon usage Cas9 gene (Methods). After 72 h, expression of sgRNA and Cas9 mRNA was verified by qPCR ( Supplementary Fig. 1 ). To test whether the RGEN disrupted the target genes we conducted SURVEYOR assays on genomic DNA isolated from transfected cells. DSB frequencies driven by each sgRNA ranged from 2.9 to 9.3% ( Fig. 1b , Supplementary Table 1 ). This assay has become the gold standard for measuring off-targets in several applications of CRISPR/Cas9, the exceptions being studies into the mechanism of action of CRISPR/Cas9 or developing improvements in the technology [19] Overall efficiencies were below values reported by other authors, reflecting our use of GX 20 sgRNA, which diminishes undesired off-target effects at the cost of cut efficiency [20] . Figure 1: Chromosomal translocation between the EWSR1 and FLI1 loci, mediated by CRISPR/Cas9 and sgRNA. ( a ) The translocation strategy. DSBs are introduced by the sgRNAs (arrowheads) mapping to introns in FLI1 (orange) and EWSR1 (turquoise). ( b ) Double-strand breaks in the targeted loci were generated by transfection of HEK293A cells with a plasmid expressing the Cas9 gene and sgRNAs E1, E2, F1 or F2. Grey arrowhead marks undigested PCR product; orange ( FLI1 ) or turquoise ( EWSR1 ) arrowheads mark digested products. Numbers on the right indicate the band sizes. The percentage of DSB is shown for each sgRNA (% indels), calculated as described in the Methods section. 293A, control non-transfected HEK293 cells. ( c ) Recovery of t(11:22) translocation after transfection with E1F2 sgRNAs. FISH analysis with the EWSR1 single-fusion probe (green, chr22; red chr11) verified reciprocal translocation (yellow signals, arrow) on representative metaphase spreads of transfected HEK293 cultures with sgRNA E1F2 and CRSIPR/Cas9. 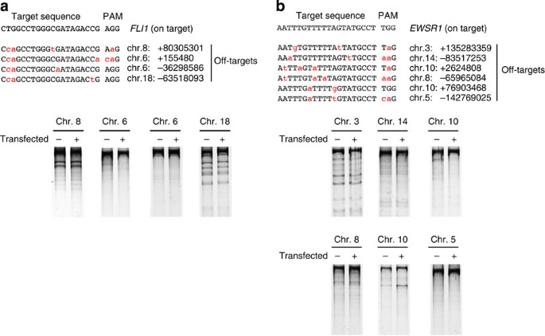Figure 2: RGEN-driven mutations at endogenous chromosomal sites. Undetectable off-target mutations for FLI1 (a) and EWSR1 (b). (Top) On-target and potential off-target sequences. Mismatched bases are shown in red. (Bottom) SURVEYOR assay comparing the cleavage efficiency at different chromosomal locations. HEK293 cells were transfected with a plasmid expressing CRISPR/Cas9 and sgRNA F2, sgRNA E1, or without sgRNA (−). For a detailed data set see Supplementary Table 2 . Scale bars represent 10 μm ( d ) Genomic PCR analysis to identify translocation breakpoint junctions. The positions of the primers used for PCR are indicated by angle symbols in the scheme in ( a ). The sequence of the amplified band is presented in the retrieved chromatogram at the bottom. 293A, non-transfected HEK293 cells. PCR control (bottom lane); detection of single copy albumin gene. ( e ) RT–PCR analysis of EWSR1–FLI1 fusion transcript expression in hygromycin-selected HEK293 cells. The positions of the primers used for PCR are indicated by angle symbols in the scheme in ( a ). The sequence of one representative clone is shown at the bottom. PCR control (bottom lane); detection of GAPDH. A673, ES cell line. ( f ) FISH analysis showing EWSR1 translocation in human MSCs. Interphase nuclei are depicted with colour probes as in ( c ). Scale bars represent 5 μm. Full size image To test whether the induced DSBs induce the reciprocal t(11;22) chromosomal translocations, we transfected HEK293A cells with four pair-wise sgRNA combinations (E1F1, E1F2, E2F1 or E2F2). At 72 h post-tranfection cell populations were screened by fluorescence in situ hybridization (FISH) with an EWSR1 single-fusion probe to detect illegitimate joining events ( Supplementary Table 1 ). Quantification in metaphase spreads and interphase nuclei revealed a reciprocal translocation rate of 1.76±0.2% ( n =3, avg±s.d. ; Supplementary Table 2 ) or the E1F2 pair-wise sgRNA combination ( Fig. 1c ), whereas none of the three other combinations scored positive for illegitimate events in 280–290 nuclei examined ( Supplementary Table 2 ). To enrich for cells harbouring the t(11;22) translocation in the E1F2-293A model, we transfected HEK293 cultures as before but with the addition of an expression plasmid encoding the hygromycin resistance gene. Screening by FISH ( Fig. 1c ) showed that after 7 days of antibiotic selection the proportion of rearranged cells was enriched to 7.7±0.8% ( n =3, avg±s.d. ; Supplementary Table 2 ). This hygromycin-selected population was used as the starting material to generate 84 derivative populations. These populations were mixed clones, derived from plating 2–10 transfected cells [21] . PCR analysis of the EWS/FLI1 DNA fusion region ( Supplementary Fig. 2 ) revealed that 37% of these 84 populations were positive for the fusion gene. Since these populations were not clonal, we performed FISH analysis to determine the percentage of translocation-positive cells within each positive population, revealing 60–80% enrichment for cells harbouring the reciprocal chromosomal translocation ( Supplementary Table 2 ). The range in the enrichment varies among the positive cell populations due to the mixed nature of each of them and the stochastic manner in which transfected and non-transfected cells were mixed. The molecular changes associated with illegitimate translocation were assessed by sequence analysis of DNA end junctions generated by DSBs. Genomic DNA from a pool of the positive clones was used as template in a PCR using primers flanking the designed DSB sequences ( Supplementary Table 1 ); a PCR band of the predicted size was retrieved from cells transfected with the E1F2 sgRNA combination ( Fig. 1d ). A DNA library for multiplexed paired-end sequencing was obtained, and deep-sequencing analysis of DNA breakpoint regions revealed robust fidelity of CRISPR/Cas9 DSB generation ( Fig. 1d and Supplementary Fig. 3 ). Scoring of the 10 best-fitting potential sequences [21] revealed no off-target mutations ( Fig. 2 ). Figure 2: RGEN-driven mutations at endogenous chromosomal sites. Undetectable off-target mutations for FLI1 ( a ) and EWSR1 ( b ). (Top) On-target and potential off-target sequences. Mismatched bases are shown in red. (Bottom) SURVEYOR assay comparing the cleavage efficiency at different chromosomal locations. HEK293 cells were transfected with a plasmid expressing CRISPR/Cas9 and sgRNA F2, sgRNA E1, or without sgRNA (−). Full size image Given the presumed mesenchymal origin of ES [22] we tested whether the CRISPR/Cas9 translocation strategy could generate the t(11;22) translocation in genetically unmodified human mesenchymal stem cells (hMSCs). Adult hMSCs were nucleofected with CRISPR/Cas9 and sgRNAs E1 and F2 as before, and the efficacy of double-strand breakage was measured by SURVEYOR assay ( Supplementary Fig. 4 ). Screening by FISH detected the presence of reciprocal t(11;22) translocation ( Fig. 1f , Supplementary Table 2 ), thus confirming the utility of the RGEN system in primary human cells, an issue of major concern [23] . Ecapitulation of gene expression changes found in Ewing’s sarcoma We next addressed whether the chromosomal translocation driven by CRISPR/Cas9 was able to replicate the synthesis of the functional fusion gene characteristic of ES. At 72 h post tranfection total mRNA from hygromycin-selected E1F2-293A cells was analysed by RT-PCR with primers flanking the breakpoint region ( Supplementary Table 1 ). After cloning the RT–PCR product, sequencing of 10 independent clones confirmed the predicted cDNA joining sequence, without error, between EWS exon 7 and FLI1 exon 5 ( Fig. 1e ). Western blot assay identified a specific antibody-reactive band in our E1F2-293A model slightly larger than the EWSR1/FLI1 protein in the ES cell line A673 ( Supplementary Fig. 5 ). The size discrepancy observed here and in the RT-PCR gel is due to the expression of the type 1 form of the chromosomal translocation the A673 ES cell line, whereas the CRISPR/Cas system generates the type 2 form. Knowing that the expression of EWSR1/FLI1 leads to significant changes in the transcription of specific genes, we tested the functionality of the fusion protein in the pool of hygromycin-selected t(11;22) positive populations. qRT–PCR on total RNA extracted 14 days post transfection confirmed the upregulation of six well-known target genes of the EWSR1/FLI1 fusion protein ( Fig. 3 ). These results suggest that the fusion protein expressed after the induction of a chromosomal translocation by the CRSIPR/Cas9 system has a similar activity to that expressed in primary ES cells. 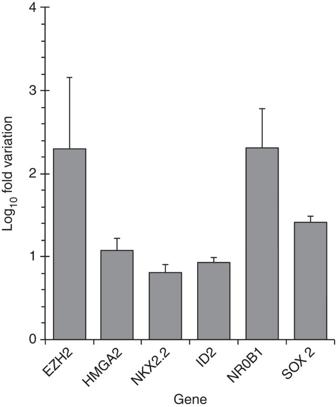Figure 3: CRISPR/Cas9-induced fusion in-frame protein EWSR1/FLI1 recapitulates transactivation properties of the natural protein. A collection of six upregulated target genes were studied by qPCR on cDNA from HEK293 cells bearing t(11:22) chromosome translocation. Data are presented as the increase above parental HEK293A. Average value of triplicates ±s.d. is shown. Figure 3: CRISPR/Cas9-induced fusion in-frame protein EWSR1/FLI1 recapitulates transactivation properties of the natural protein. A collection of six upregulated target genes were studied by qPCR on cDNA from HEK293 cells bearing t(11:22) chromosome translocation. Data are presented as the increase above parental HEK293A. Average value of triplicates ±s.d. is shown. Full size image Induction of the AML t(8;21) chromosomal translocation To test the general applicability of the CRISPR/Cas9 system for in vitro induction of human chromosomal translocations, we assessed its ability to trigger the t(8,21)(q22;q22) chromosomal translocation frequently found in AML. The result of this translocation is an in-frame fusion of the 5′ region of the RUNX1 gene with almost the entire ETO gene [24] . HEK293A cells were co-transfected with pair-wise combinations of sgRNAs complementary to the intron sequences at ETO intron 1 (Et1, Et2) and RUNX1 intron 5 (R1, R2) [25] ( Supplementary Table 1 ) and the CRISPR/Cas9 expression cassette ( Fig. 4a ). SURVEYOR assay analysis of PCR-amplified genomic DNA from transfected and non-selected cultures revealed 8.7–25% efficiency of double-strand breakage ( Fig. 4b ). FISH analysis with a double-fusion probe revealed illegitimate junctions in 0.96±0.1 to 4.07±0.3% ( n =3, avg±s.d. ; Supplementary Table 2 ) of transfected cells, depending on the combination of sgRNAs used ( Fig. 4c , Supplementary Table 2 ). Molecular analysis of the breakpoint junctions confirmed that accurate DNA-end joining was taking place ( Fig. 4d and Supplementary Fig. 6 ), and RT–PCR analysis of mRNA confirmed expression of the RUNX1/ETO fusion gene derived from the chromosomal translocation ( Fig. 4e ). To characterize the ability of the system to support disease translocations in primary cells we assessed the generation of the RUNX1/ETO translocation in CD34+ human haemopoietic/progenitor stem cells (HPSCs) isolated from umbilical cord blood (CB). FISH analysis showed that the t(8,21) translocation was produced in human HPSCs nucleofected with the CRISPR/Cas9-encoding plasmid and sgRNA R1/Et2 ( Fig. 4f , Supplementary Table 2 ). 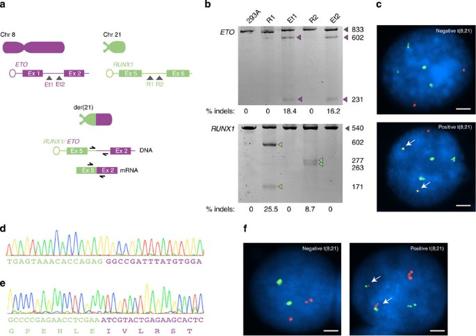Figure 4: Chromosomal translocation between theAML-1andETOloci, mediated by CRISPR/Cas9 and sgRNA. (a) The translocation strategy. DSBs are introduced by the sgRNAs (arrowheads) mapping to introns inETO(purple) andRUNX1(green). (b) DSB efficiency in theRUNX1/ETOtargeted sequence for each sgRNA studied. Double-strand breaks in the targeted loci introduced by CRISPR/Cas9 in HEK293 cells co-transfected with sgRNAs R1, R2, Et1 or Et2. Grey arrowhead marks undigested PCR product; purple (ETO) or green (RUNX1) arrowheads mark digested PCR products. Numbers on the right indicate the band sizes. The percentage of DSBs is shown for each sgRNA (% indels) calculated as described in the Methods section. 293A, non-transfected HEK293 cells. (c) Recovery of t(8:21) translocation after selection of transfected HEK293 cells with R1Et2 sgRNAs. FISH analysis using theRUNX1/ETOdouble-fusion probe (green, chr21; red chr8) verified the reciprocal translocation (yellow signals). (d) Genomic PCR analysis to identify translocation breakpoint junctions. The positions of the primers used for genomic PCR are indicated by angle symbols in the scheme in (a). The sequence of the amplified band is presented in the retrieved chromatogram at the bottom. (e) Expression of the fusionRUNX1/ETOfusion transcript in hygromycin-selected HEK293 cells. The chromatogram sequence of one representative clone of six retrieved clones is shown, illustrating the accurate breakpoint joining in the RNA expressed from the translocated chromosome. Primers used for PCR are indicated by angle symbols in the scheme in (a). (f) FISH analysis of chromosome 8 (red) and 21 (green), verifying reciprocal chromosomal translocation in CD34+ human haematopoietic stem cells. Scale bars represent 5 μm. Figure 4: Chromosomal translocation between the AML-1 and ETO loci, mediated by CRISPR/Cas9 and sgRNA. ( a ) The translocation strategy. DSBs are introduced by the sgRNAs (arrowheads) mapping to introns in ETO (purple) and RUNX1 (green). ( b ) DSB efficiency in the RUNX1/ETO targeted sequence for each sgRNA studied. Double-strand breaks in the targeted loci introduced by CRISPR/Cas9 in HEK293 cells co-transfected with sgRNAs R1, R2, Et1 or Et2. Grey arrowhead marks undigested PCR product; purple ( ETO ) or green ( RUNX1 ) arrowheads mark digested PCR products. Numbers on the right indicate the band sizes. The percentage of DSBs is shown for each sgRNA (% indels) calculated as described in the Methods section. 293A, non-transfected HEK293 cells. ( c ) Recovery of t(8:21) translocation after selection of transfected HEK293 cells with R1Et2 sgRNAs. FISH analysis using the RUNX1/ETO double-fusion probe (green, chr21; red chr8) verified the reciprocal translocation (yellow signals). ( d ) Genomic PCR analysis to identify translocation breakpoint junctions. The positions of the primers used for genomic PCR are indicated by angle symbols in the scheme in ( a ). The sequence of the amplified band is presented in the retrieved chromatogram at the bottom. ( e ) Expression of the fusion RUNX1/ETO fusion transcript in hygromycin-selected HEK293 cells. The chromatogram sequence of one representative clone of six retrieved clones is shown, illustrating the accurate breakpoint joining in the RNA expressed from the translocated chromosome. Primers used for PCR are indicated by angle symbols in the scheme in ( a ). ( f ) FISH analysis of chromosome 8 (red) and 21 (green), verifying reciprocal chromosomal translocation in CD34+ human haematopoietic stem cells. Scale bars represent 5 μm. Full size image The aetiology of human neoplasias often involves chromosomal translocations, and models mimicking this feature are essential for understanding the determinants of malignancy. Several strategies have been used to generate cellular and animal models, including transgenesis of the fusion gene of interest or the generation of an ‘artificial’ fusion gene through the introduction of a cDNA element into an intron target gene [26] . However, the most faithful recapitulation of the reciprocal translocations found in human neoplasias is the experimental generation of an interchromosomal reciprocal translocation. Cre/loxP, TALENs and ZFNs technologies have already been used to achieve this, demonstrating that it is possible to reproduce cancer-relevant translocations [4] , [5] , [6] . However, the complexity of the design, the complexity of the method and, more importantly, the extremely low frequencies obtained—averaging below 10 −3 —limit applicability of these methods. In the present study, we show that the CRISPR–Cas9 system can be easily adapted for the generation of chromosomal translocations in human cultured cell lines and primary adult stem cells. Moreover, the chromosomal translocation in the ES leads to overexpression of the same set of genes that is consistently increased in primary samples from patients. FISH analysis provided an accurate measure of the efficiency of the chromosomal translocations induced by the CRISPR/Cas9 system, and showed that the cell frequencies of chromosomal translocation ( Supplementary Table 2 ) are three to four log-units higher than those obtained with other methods based on nucleases and recombinases [5] , [6] , [27] . The method also enjoys the benefits common to other CRISPR–Cas9 techniques, in being cheap, simple, easy and intuitive to design, and reliable. This makes for a highly efficient process, allowing cell clones with the desired chromosomal translocation to be selected by screening a few hundred transfected cells. These features might make RGEN the tool of choice for generating cellular or animal models of the human chromosomal translocations that cause many cancers. Little is known about the precise molecular mechanisms by which chromosomal translocations are generated in vivo . The process consists of two DNA DSBs followed by a joining of the resulting DNA ends in a new configuration. The translocations are likely mediated by the non-homologous end joining (NHEJ) DSB repair pathway, though to date it is not clear whether this involves the canonical or alternative pathways [23] . It is known that NHEJ does not require any homology to repair a DSB; however, a few nucleotides of terminal microhomology are often utilized by the NHEJ enzymes if present, leading in this case to an error-prone repair associated with deletions at the repair junctions. Sequencing of leukaemia patient samples revealed that translocation junctions often have deleted sequences, indicating that these translocations predominantly arose by this mechanism. Deep-sequencing analysis of the junction regions in our models generated using the CRISPR/Cas9 system revealed minor variations. This might appear surprising, compared with the chromosomal translocations generated in human tumour cells. However, it is important to keep in mind that the CRISPR–Cas9 approach is a nuclease system that induces blunt-ended DSBs. A recent report suggests that the repair of signal joints, which results from the direct ligation of blunt ends, is largely error-free [28] . The authors also indicate that the accuracy of the repair is dictated by the structure of the DNA ends rather than by the NHEJ machinery. Although our experiments were not designed to address such processes, our results suggest that the end joining of blunt-ended DSBs by the NHEJ machinery might be the main process involved in the repair mechanism by which the CRISPR–Cas9 system generates chromosomal translocations [23] . The lack of suitable methodologies has made it difficult to establish the factors involved and the time-line followed by the chromosomal translocations that cause most leukaemia and sarcoma malignancies. With further optimization, the CRISPR–Cas9-based tool presented here has the potential to generate models that will facilitate study of the step-wise events that drive these tumours. RGEN-based methods like the one we describe here may also make large-scale studies into the aetiology of these malignancies more affordable. Mammalian cell culture Experiments in this study were conducted with the HEK cell line HEK293A (CRL-1573, American Type Culture Collection (ATCC), USA), umbilical-cord-derived mesenchymal stem cells (hMSCs, PCS-500-010, ATCC), the A673 cell line (CRL-7910, ATCC) and umbilical CB CD34+ cells. HEK293A and A673 cells were cultured under standard conditions in Dulbecco’s modified Eagle’s medium (Lonza, Spain) supplemented with 1% Glutamax (Life Technologies, Spain), 10 mg ml −1 antibiotics (penicillin and streptomycin, Gibco, Life Technologies) and 10% fetal bovine serum (FBS; (Gibco, Life Technologies). hMSCs were cultured in MesenPRO RS Medium (Gibco, Life Technologies). Human CB was collected and used within 12 h according to institutional guidelines. All procedures were approved by the Ethical Research and Animal Care Committee of the Institute of Health Carlos III (CEI PI 32_2009). Low-density mononuclear cells were isolated from CB diluted 1:2 in PBS by centrifugation in Histopaque-1077 (SIGMA Diagnostics, USA). Haematopoietic progenitor/stem cells were purified by separation on two sequential CD34 MicroBead MACS columns (Miltenyi Biotec, Germany). CD34+ cells were cultured in Iscove’s modified Dulbecco’s medium containing 20% FBS, 100 mg ml −1 penicillin–streptomycin and a cytokine cocktail of FLT3L (100 ng ml −1 ), SCF (100 ng ml −1 ), TPO (100 ng ml −1 ), IL-6 (20 ng ml −1 ), GM-CSF (20 ng ml −1 ), EPO (6 U ml −1 ) and IL-3 (50 ng ml −1 ; Peprotech, UK). All cells were cultured at 37 °C in a humidified incubator in a 5% CO 2 , 20% O 2 atmosphere. Construction of Cas9-encoding plasmids The human codon-usage-optimized Cas9-coding sequence (4,140 bp), derived from Streptococcus pyogenes strain M1 GAS (NC_002737.1), was obtained from Addgene (no. 41815). The Cas9-encoding DNA segment was subcloned into pLV, which was derived from pLVX shRNA2 (Clontech), and the chimeric sequences were synthesized (IDT, USA) and cloned in the same backbone. In this vector, the Cas9 protein is expressed under the control of the SFFV promoter and the sgRNA is cloned under the control of a U6 promoter. Expression of Cas9 RNA in HEK293A cells was confirmed by qPCR ( Supplementary Fig. 1 ), using the primers detailed in Supplementary Table 1 . Transfection and electroporation Cells were transfected with endotoxin-free DNA (Qiagen, Spain) and transfections were carried out in six-well plates (BD Biosciences, USA). For the calcium phosphate method cells were transfected as previously described [29] . Briefly, the day before transfection 500,000 HEK293A cells were seeded in each well, and under a confluence of ~80–90% the transfection was carried out the following day. A total amount of 6 μg of plasmid DNA was prepared, adding 30 μl of CaCl 2 (2.5 M) in a final amount of 250 μl of milliQ water; in parallel, 250 μl of an HBS 2 × solution was prepared and both tubes were mixed. Finally, the transfection mix was added in a drop-wise manner to the cells, allowed to stay in the incubator for 4–6 h and finally the medium was changed. After 48–72 h, the cells were processed properly for the subsequent analysis. For electroporation, we employed the Neon transfection System (Invitrogen, Life Technologies, USA). Protocols hMSC, PBMC and HL-60 were adapted from the repository database of the manufacturer with minimal modifications. Briefly, hMSCs were electroporated at an 80–90% density. Cells were trypsinized and washed with DPBS twice, counted and resuspended in R solution (both from Invitrogen, Life Technologies). Tips of 10 μl size were used to electroporate 50,000–100,000 cells using a 40-ms single pulse of 990 V. Next, cells were seeded in a 12-well plate. The following day, the media was replaced with fresh MesenPRO media. In the case of CD34+ cells, 200,000 cells were electroporated with 10-μl tips using a 20 ms single pulse of 2,150 V. Antibiotic selection was performed at 72 h post transfection using media supplemented with the selective agent. HEK293 and MSC cells were selected using hygromycin (Sigma, USA) at concentrations of 100 and 40 μg ml −1 , respectively. CD34 cells were selected using puromycin at a concentration of 0.25 μg ml −1 . Genomic DNA extraction and standard PCR analysis Genomic DNA was extracted using standard procedures. Briefly, 5–10 × 10 6 cells were either trypsinized or scraped, washed in PBS, pelleted and lysed in 100 mM NaCl, 50 mM Tris (pH 8.0), 100 mMEDTA and 1% SDS. After overnight digestion at 56 °C with 0.5 mg ml −1 of proteinase K (Roche Diagnostics, USA), the DNA was cleaned by saturated NaCl precipitation and the clear supernatant precipitated with isopropanol, washed with 70% ethanol, air-dried and resuspended overnight at room temperature in 1 × TE. Serial dilutions of the DNA were quantified with a NanoDrop ND 1000 Spectrophotometer (NanoDrop Technologies, Spain). Standard PCR was performed in a Veriti 96-well Thermal Cycler system (Applied Biosystems, USA) at the following conditions: template denaturation at 95 °C for 1 min, followed by 30 cycles of denaturation at 94 °C for 30 s, annealing at 62.5 °C for 30 s, and extension at 72 °C for 60 s, and a final extension of 5 min at 72 °C. The primers used are summarized in Supplementary Table 1 . RNA extraction and PCR Total RNA was extracted from tissues and cell cultures using Trizol (Sigma-Aldrich, USA), followed by treatment with RNase-free DNAse (Roche Applied Science, Spain). cDNA was synthesized from 500 ng of total RNA using the Superscript III First Strand cDNA Synthesis Kit (Life Technologies). Specific mRNAs were quantified by qRT-PCR using an ABI Prism 7900 HT Detection System (Applied Biosystems, Foster City, CA, USA) and SYBR green detection. PCR was performed in 96-well microtest plates with SYBR Green Master Mix (Applied Biosystems) for 40 cycles. In all experiments, mRNA amounts were normalized to the total amount of cDNA by using amplification signals for hGUSB and GAPDH . Each sample was determined in triplicate, and at least three independent samples were analysed for each experimental condition. For RT–PCR experiments, 1 μg of total RNA was reverse-transcribed with the Superscript III First Strand cDNA Synthesis Kit (Life Technologies). PCR amplification was performed using Taq DNA Polymerase (Roche Diagnostics, USA). The amplification profile consisted of 40 cycles of denaturation at 94 °C for 30 s, annealing at 60 °C for 50 s and elongation at 72 °C for 50 s. PCR products were identified by gel electrophoresis. Positive and negative controls were performed at all steps. The amplification primers for the EWS/FLI1 and RUNX1/ETO fusion transcripts are summarized in Supplementary Table 1 . Western blot Proteins were extracted by standard procedures in the presence of Complete Protease Inhibitor Cocktail Tablets (Roche Applied Science, USA). Western blots were carried out by standard methods on proteins transferred to PVDF using TransFi (Invitrogen, Life Technologies). Membranes were probed for EWS/FL1 with monoclonal mouse anti-human FLI-1 antibody (1/500; BD Pharmingen, USA) or for GAPDH (AbCam, Cambridge, UK), with antibodies diluted 1/2,500 in PBS/0.1% Tween-20 (PBS-T). Secondary antibodies were HRP-conjugated with goat anti-mouse IgG (1/1,000) and goat anti-Rabbit (1/500; Dako, Barcelona, Spain), and blots were developed with ECL (GE Healthcare, Alcobendas, Spain). Fluorescence in situ hybridization Two sets of probes were used to detect EWS/FLI1 and RUNX1/ETO chromosomal translocations. Specific bacterial artificial chromosomes (BAC) for the EWSR1 and FLI1 genes (RPCI-11 Human BAC Clone Library, Children’s Hospital Oakland Research Institute (CHORI)) were directly labelled with FITC or Texas-Red fluorochromes by nick translation (Vysis, London, UK) according to the manufacturer’s specifications. These BACs were used to detect the EWS/FLI1 rearrangement. The LSI AML1/ETO Dual Colour, Dual Fusion Translocation Probe (Vysis, Abbott Molecular, USA) was used to detect the t(8;21) chromosomal translocation. Chromosome spreads, prepared directly from transfected HEK293A cells, were left overnight at room temperature. Slides were placed on a plate at 90 °C for 10 min, dehydrated through a series of ethanol washes, and denatured in the presence of a probe on a plate at 75 °C for 1 min. After post-hybridization washes, the chromosomes were counterstained with DAPI in Vectashield mounting medium (Vector Laboratories, USA). Cell images were captured using a charge-coupled device camera (Photometrics SenSys camera) connected to a computer running the Chromofluor image analysis system (Cytovision, Applied Imaging Ltd, UK). Library preparation, sequencing and primary data processing PCR DNA bands were purified using the QIAquick Gel Extraction Kit (Qiagen) and used as the template for a library preparation. DNA size selection after a fragmentation by acoustic shearing on a Covaris S2 instrument was set to 50 bp. The sequencing library was prepared using oligonucleotides (Illumina), enzymes (Enzymatics) and manual purification between each enzymatic reaction by column-based methods (Qiagen). Brieftly, DNA fractions of 50 bp were ligated to Illumina’s adapters and enriched by amplifying with the Phusion high-fidelity polymerase (New England Biolabs) using Illumina PE 1.0 and 2.0 primers, and index primers (Illumina). The resulting purified DNA libraries were quantified via electrophoretic separation on a microfluidics platform, and sequenced using the Illumina Genome Analyzer IIx in a single-read format by following the manufacturer’s protocols. Analysis, per-cycle base calling and quality score assignment were performed with Illumina Real Time Analysis software. Illumina BCL files were converted to bam format with the Illumina2bam tool (Wellcome Trust Sanger Institute). SURVEYOR assay and off-target detection The SURVEYOR Nuclease Kit (Transgenomic, Durvit, Spain) was used to determine Cas9-mediated cleavage efficiency. After transfection or electroporation, cells were maintained for 72 h in a humidified incubator. Genomic DNA was extracted, and the flanking region of each guided RNA sequence and its possible off-targets were PCR-amplified (target sites and primers are listed in Supplementary Table 1 ). Each product was confirmed by gel electrophoresis and further purified on a Qiaquick Spin Column (Qiagen). A total of 350 ng of each PCR product was further reannealed (in NEB Buffer 2, NEB) in 20 μl final volume, in order to form heteroduplexes. After that, products were processed with the SURVEYOR Nuclease Kit and analysed in TBE 10% polyacrylamide gels (Bio-Rad, USA). Gels were stained with SYBR Gold (Life Technologies) for 20 min and washed with TBE 1 × for 25 min. Images were acquired with the Gel Doc imaging system (Bio-Rad), and relative band intensities were quantified with ImageLab (BioRad). NHEJ frequency was quantified using the formula 100 × (1−(1− a /( a + b ))1/2), where a is the band intensity of the cleavage products and b is the band intensity of the uncleaved PCR product. How to cite this article: Torres, R. et al . Engineering human tumour-associated chromosomal translocations with the RNA-guided CRISPR–Cas9 system. Nat. Commun. 5:3964 doi: 10.1038/ncomms4964 (2014). The funders had no role in study design, data collection and analysis, decision to publish or preparation of the manuscript.